Role of domain walls in the abnormal photovoltaic effect in BiFeO3 Recently, the anomalous photovoltaic (PV) effect in BiFeO 3 (BFO) thin films, which resulted in open circuit voltages ( V oc ) considerably larger than the band gap of the material, has generated a revival of the entire field of photoferroelectrics. Here, via temperature-dependent PV studies, we prove that the bulk photovoltaic (BPV) effect, which has been studied in the past for many non-centrosymmetric materials, is at the origin of the anomalous PV effect in BFO films. Moreover, we show that irrespective of the measurement geometry, V oc as high as 50 V can be achieved by controlling the conductivity of domain walls (DW). We also show that photoconductivity of the DW is markedly higher than in the bulk of BFO. Recently, the entire field of photoferroelectrics has been revitalized by reports of an abnormal photovoltaic (PV) effect in BiFeO 3 (BFO) thin films [1] . The main characteristics of this abnormal PV effect are very large open circuit photovoltages ( V oc ) exceeding the band gap of the material. For instance, in high quality BFO thin films, V oc is several times larger than the band gap (~2.7 eV). However, reports on the PV effect in different BFO systems are rather contradictory. In a specific in-plane geometry of measuring electrodes with respect to the domain pattern, films with periodic ferroelectric/ferroelastic stripe domain patterns show V oc values above [1] or below the band gap [2] . In the normal plane-parallel capacitor geometry, the measured V oc value has always been below the band gap values [3] , [4] . Single crystals show, or do not show, large V oc values depending on the source or perhaps the crystal growth details [5] , [6] , [7] . To the best of our knowledge, there is not yet any report of abnormal PV effect in BFO ceramics. In the original report on the abnormal PV effect on epitaxial BFO films, it was shown that V oc values as large as 15 V can be obtained, but only in a specific geometry when the ferroelectric/ferroelastic domain walls (DW) are running parallel to the macroscopic electrodes. If the ferroelectric domains are perpendicular to the electrodes, there was no sizable PV effect, but only a photoconductive effect was detected [1] . This has led to the hypothesis that the abnormal PV effect in BFO originates solely in the DW by the following mechanism: the photogenerated electron-hole pairs within the domain wall are separated by the strong field existing in this region, whereas within the bulk of the domains, the carriers will strongly recombine. The separated electrons and holes will accumulate only at the DW, building in such a way a small voltage across each domain wall. These voltages, although in the mV range, will sum up over macroscopic distances leading to the large open circuit voltage [8] . The bulk photovoltaic (BPV) effect, which is known to exist in materials lacking inversion symmetry such as LiNbO 3 , BaTiO 3 or Pb(Zr,Ti)O 3 (refs 9 , 10 , 11 , 12 , 13 , 14 ), was a priori ruled out. Subsequent experiments have shown that generation and recombination of photogenerated carriers in BFO single crystals are primarily affected by the presence of shallow energy levels, and that DW are not having a major role in the corresponding PV effect. Moreover, the photoexcited carriers are generated across the entire crystal, the recombination of these carriers is rather uniform and it is not necessarily stronger within the domains compared with the vicinity of the DW [5] , [15] . We show here that the abnormal PV effect in BFO thin films with open circuit voltages ( V oc ) as large as 50 V exists irrespective of the domain wall geometry and that the DW are having a rather different role than initially proposed. We confirm that the abnormal PV effect in BFO is due to the BPV effect, as recently predicted by ab initio calculations using the ‘shift currents’ concept, which have been able to predict the short-circuit photocurrent, viz. magnitude and even spectral features, demonstrating that these shift currents should dominate the BPV response in BFO [16] , [17] . Thin film fabrication Nominally 100-nm thick (001)-oriented BFO epitaxial films were deposited by pulsed laser deposition on (110)-oriented TbScO 3 . Details on film growth and structure are given in the Methods section and Supplementary online Material (SOM) ( Supplementary Figs S1–S3 ). Samples showing stripe domains comprising either 109° or 71° domain boundaries have been fabricated by choosing the growth conditions. In case of 109° domains, the stripes run along [100] c whereas in 71° domains, stripes run along the [010] c direction. 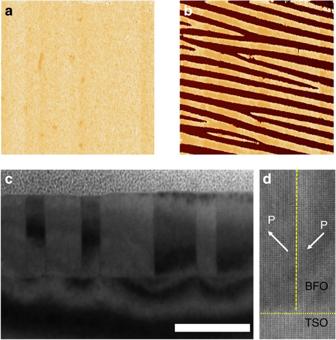Figure 1: Domain configurations. PFM images (3.5 × 3.5 μm scan) of pristine sample with 71° domains, (a) out-of-plane phase image (b) in-plane phase image showing stripes, which run along [010]c. (c) Two-beam bright-field TEM image of a BFO epitaxial film grown on TbScO3taken with near g=001c. The dark and bright contrasts show the domain structure of the BFO thin film. The type of domains was identified as 109° stripe domains with (100)cvertical DW. Scale bar, 100 nm. (d) The high-resolution TEM image corresponding toFig. 1cshows coherency on either side of the vertical domain wall and the two polarization variants. Figure 1 shows the corresponding piezoforce microscope (PFM) images of the stripe domain pattern obtained on the thin films with 71° domains and a cross-sectional TEM image of a sample with dominant 109° domains. Figure 1: Domain configurations. PFM images (3.5 × 3.5 μm scan) of pristine sample with 71° domains, ( a ) out-of-plane phase image ( b ) in-plane phase image showing stripes, which run along [010] c . ( c ) Two-beam bright-field TEM image of a BFO epitaxial film grown on TbScO 3 taken with near g=001 c . The dark and bright contrasts show the domain structure of the BFO thin film. The type of domains was identified as 109° stripe domains with (100) c vertical DW. Scale bar, 100 nm. ( d ) The high-resolution TEM image corresponding to Fig. 1c shows coherency on either side of the vertical domain wall and the two polarization variants. Full size image Platinum electrodes of 250 μm length and variable interelectrode distances (from 15 μm up to 100 μm) were fabricated by sputter deposition using conventional photolithography and lift-off technique. Devices were aligned parallel and perpendicular to the DW, as shown schematically in Fig. 2 (also Supplementary Fig. S4 ). The photoelectric effect was measured by illuminating the gap between the electrodes with a 405 nm ( hυ = 3.06 eV) laser with a maximum power of 80 mW and simultaneously measuring the photocurrent using a high-input impedance electrometer. 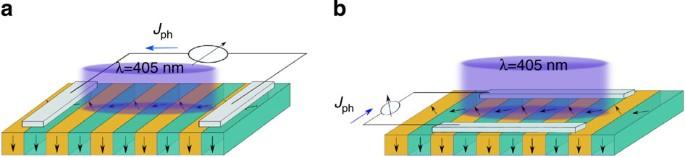Figure 2: Measurement geometries. Schematic showing the patterned electrodes on top of a film with majority 71° domains (not to scale) and typical measurement geometries in which the electrodes are running: (a) parallel (PLDW) and (b) perpendicular to DW (PPDW), respectively. The arrows indicate the direction of polarization in out-of-plane (up–down) and in-plane (left–right) directions. Figure 2: Measurement geometries. Schematic showing the patterned electrodes on top of a film with majority 71° domains (not to scale) and typical measurement geometries in which the electrodes are running: ( a ) parallel (PLDW) and ( b ) perpendicular to DW (PPDW), respectively. The arrows indicate the direction of polarization in out-of-plane (up–down) and in-plane (left–right) directions. Full size image Abnormal PV effect To get a better insight into the actual mechanism of the abnormal PV effect in BFO, we have performed detailed photoelectric investigations on BFO epitaxial thin films with periodical domain patterns of 109° and 71° DW, respectively. At room temperature (RT) both geometries, parallel to the DW (PLDW) and perpendicular to the DW (PPDW), show PV behaviour similar to previous reports for 109° DW [2] . Current voltage (IV) characteristics under illumination shown in Fig. 3 reveal V oc values larger than the band gap of BFO (5 V for an interelectrode gap of 100 μm) in the PLDW geometry and nearly zero for the DW running perpendicular to the electrodes. Surprisingly, the BFO sample comprising 71° DW shows at RT a sizable V oc in both configurations, viz. −6.6 V perpendicular to the DW (PPDW) and − 7.6 V parallel to the DW (PLDW), as shown in Fig. 3b . 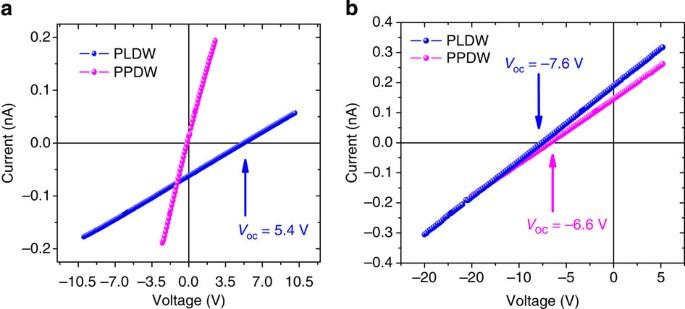Figure 3: Abnormal PV effect. I-V characteristics under illumination with monochromatic light (hυ=3.05 eV) of BFO thin films comprising (a) 109° and (b) 71° periodic stripe domains. Figure 3: Abnormal PV effect. I-V characteristics under illumination with monochromatic light ( hυ =3.05 eV) of BFO thin films comprising ( a ) 109° and ( b ) 71° periodic stripe domains. Full size image Temperature-dependent V OC Photoelectric measurements were conducted at temperatures ranging from 80 to 450 K. By performing the analysis at different temperatures down to 80 K, we notice that in both geometries and DW variants by decreasing the temperature well below room temperature, the V oc values increase dramatically, that is, for 109° domains to more than 17 V and for 71° domains to more than 50 V, as shown in Fig. 4 . The temperature dependence of V oc has a similar behaviour for both geometries; it increases at low temperature to values that are in both cases well above the band gap with an obvious increase at temperatures lower than 200 K. The most dramatic increase of V oc to about 20 times the bang gap is for 71° DW. For 109° domains in the PPDW geometry, the open circuit voltage, which at RT was almost zero, becomes at 83 K as large as 12 V. At RT, in the case of 71° domains in the PPDW geometry, where according to the initial model the open circuit voltage should be below the band gap, the V oc values are larger than 5 V. The sizable V oc in the perpendicular geometry in the case of 71° domains at RT and the dramatic increase of V oc with decreasing temperature in all cases suggest that those mechanisms in which the DW are at the origin of this effect, as it has been previously assumed [1] , [8] , are not valid and both bulk and DW should have a different role. 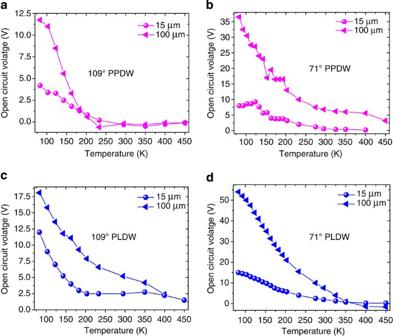Figure 4: Temperature-dependentVoc. Temperature dependence of the open circuit voltage for 109° DW in (a) perpendicular and (c) parallel geometry and for 71° DW in (b) perpendicular and (d) parallel geometry for two gap widths, that is, 15 μm and 100 μm. Figure 4: Temperature-dependent V oc . Temperature dependence of the open circuit voltage for 109° DW in ( a ) perpendicular and ( c ) parallel geometry and for 71° DW in ( b ) perpendicular and ( d ) parallel geometry for two gap widths, that is, 15 μm and 100 μm. Full size image Bulk PV effect Keeping in perspective the temperature-dependent behaviour of V oc , the only viable alternative explanation for the anomalous PV effect in BFO remains the BPV or photogalvanic effect, as known for materials lacking inversion symmetry, discovered by Chynoweth [9] and later analysed theoretically by others [18] , [19] . Accordingly, under uniform illumination, the photocurrent J ph is due to an asymmetric generation in k -space, and under open circuit conditions, the open circuit voltage ( V oc ) is given by: where ρ is the resistivity and L is the distance between the electrodes. Moreover, according to Fridkin [13] , V oc scales inverse proportionally with both dark conductivity and photoconductivity, so that equation (1) becomes: where σ d and σ ph are dark conductivity and photoconductivity, respectively. 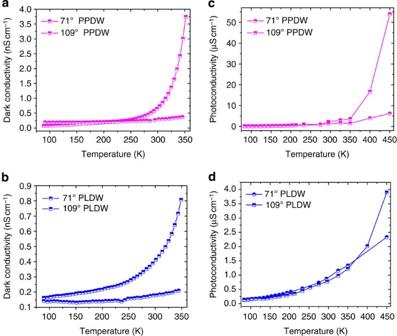Figure 5: Conductivity measurement. Temperature dependence of dark conductivity (a,b) and photoconductivity (c,d) measured with the electrodes running perpendicular (PPDW) and parallel (PLDW) to the DW for both 109° and 71° domains. The exponential-like increase of V oc with decreasing temperature is corroborated by the temperature variation of both dark conductivity and photoconductivity shown in Figure 5 , which represents a direct proof of (1) and (2) for the case of BFO thin films. Figure 5: Conductivity measurement. Temperature dependence of dark conductivity ( a , b ) and photoconductivity ( c , d ) measured with the electrodes running perpendicular (PPDW) and parallel (PLDW) to the DW for both 109° and 71° domains. Full size image As it can be easily seen, both dark and photoconductivity are higher in the case of 109° domains when compared with 71° domains. Also, both dark and photoconductivity are higher in the perpendicular than in the parallel geometry. These observations imply first that the DW have an enhanced conductivity and are largely governing both the dark and photoconductivity of the BFO films. This is not surprising, as the dc dark conductivity of 109° DW has been already estimated to be at least four orders of magnitude higher than the bulk of BFO [20] . In the same time, the conductivity of 71° DW is lower compared with the 109° DW, which is also in agreement to previous results [21] . To explain the existence and/or absence of the abnormal PV effect and respectively a value of the open circuit voltage ( V oc ) larger than the band gap, we can assume that a photocurrent is rather uniformly generated in the entire film by the photogalvanic effect or, as recently shown using ab initio calculation, by so called ‘shift currents’ [16] . In the same time the open circuit voltage is established according to (2) by the actual conductivity of the BFO film considering both the bulk and the domain wall conductivity. The effective sample conductivity is given by a simple equivalent circuit, which is either parallel or serial, depending on the geometrical arrangement of the collecting electrodes relative to the DW. As schematically shown in Fig. 6 , in the perpendicular geometry (PPDW), the equivalent circuit is a parallel circuit and the effective conductivity is given by the sum of both bulk and domain wall conductivities σ total =(σ bulk +σ DW ), whereas in the parallel geometry (PLDW), the appropriate equivalent circuit is the series circuit and in this case, the inverse of the effective conductivity is the sum of the inverse conductivities (σ total ) −1 =(σ bulk ) −1 +(σ DW ) −1 . 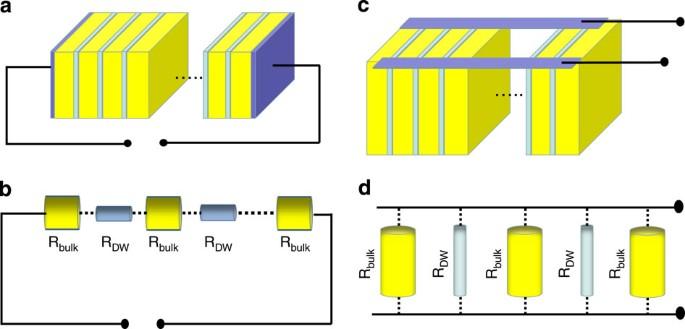Figure 6: Two resistance model. A schematic showing the periodic arrangement of domains and DW in BFO thin films for the (a) parallel (PLDW) and (c) perpendicular (PPDW) geometry with respect to the DW. An equivalent circuit considering that the domain bulk and DW have different resistances, Rbulkand RDW, is shown for both the geometries in (b) PLDW and (d) PPDW. Figure 6: Two resistance model. A schematic showing the periodic arrangement of domains and DW in BFO thin films for the ( a ) parallel (PLDW) and ( c ) perpendicular (PPDW) geometry with respect to the DW. An equivalent circuit considering that the domain bulk and DW have different resistances, R bulk and R DW , is shown for both the geometries in ( b ) PLDW and ( d ) PPDW. Full size image According to this simple model, the effective resistance is lower when the DW are running perpendicular to the electrodes and thus, the open circuit voltage should be lower in the PPDW geometry. This is valid for all cases (see Fig. 5 ). For 109° domains in which the DW are much more conductive than in 71° domains, the V oc for all the cases was lower than what was measured in cases with 71° domains. BPV effect in BFO films In order to prove the existence of the bulk PV effect (BPV) in our films, we measured the PV current for all the systems by changing the angle between the plane of the linearly polarized light and the direction of current flow. The BPV effect has been studied extensively in non-centrosymmetric materials like KNbO 3 , BaTiO 3 , reduced LiTaO 3, so on. The BPV effect in ferroelectrics can be expressed in the form of an equation given by [14] where β ijk is a third rank BPV tensor and I is the intensity of light. According to equation (3), when a homogenous ferroelectric crystal is illuminated uniformly by a linearly polarized light, it leads to the generation of a PV current . The behaviour of this PV current in terms of its sign and magnitude depends on the orientation of the crystal with respect to the projections of the electric field of the linearly polarized light onto the plane of the sample along X and Y directions, namely and . 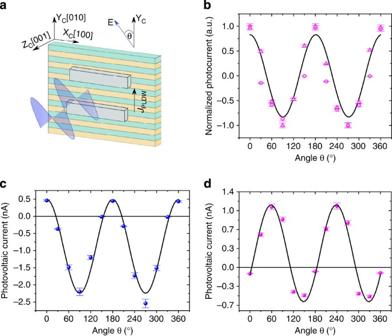Figure 7: BPV effect. (a) Schematic of a sample showing stripes, which represent the DW either of the 109° or 71° stripe domain system. The coordinate system is given by XYZ. The schematic shows how the vectorEof the linearly polarized light is aligned with the direction of the current flowJfor the PLDW case. (b) Normalized PV current measured at different angles (θ), which the polarization axis of the linearly polarized light makes with the direction of the current flow in the PLDW geometry for samples with 71° (circle) and 109° (triangle) domains, respectively. The solid line represents the fit with equation (4). PV current measured and predicted by varying the angleθthat the light polarization axis makes with the direction of current flow inc) PLDW geometry andd) PPDW geometry for a film consisting of 71° domains. In all, the plots a 5% (rough estimate) error has been incorporated in the PV current measurement to compensate for any misalignment in laser beam spot positioning. Based on equation (3), and as detailed in the Methods, the current generated along the two orthogonal directions X and Y with the light propagating along the Z direction is given by [14] , [22] , [23] , [24] Figure 7a depicts the arrangement of the setup in which the coordinate system shown follows the pseudo-cubic notation of the BFO film so that the direction X is given by [100], Y is given by [010] and Z is given by [001]. The light illumination is along the Z [001] direction. For these measurements, the angle θ=0° means that the E vector of the linearly polarized light is parallel to the direction of the current flow, whereas an angle of 90° means that E is perpendicular to the current flow direction. The normalized values for the measured PV current by varying the angle between the current direction and the polarization axis of the light are presented in Fig. 7b . Figure 7: BPV effect. ( a ) Schematic of a sample showing stripes, which represent the DW either of the 109° or 71° stripe domain system. The coordinate system is given by XYZ. The schematic shows how the vector E of the linearly polarized light is aligned with the direction of the current flow J for the PLDW case. ( b ) Normalized PV current measured at different angles ( θ ), which the polarization axis of the linearly polarized light makes with the direction of the current flow in the PLDW geometry for samples with 71° (circle) and 109° (triangle) domains, respectively. The solid line represents the fit with equation (4). PV current measured and predicted by varying the angle θ that the light polarization axis makes with the direction of current flow in c ) PLDW geometry and d ) PPDW geometry for a film consisting of 71° domains. In all, the plots a 5% (rough estimate) error has been incorporated in the PV current measurement to compensate for any misalignment in laser beam spot positioning. Full size image It is rather evident from the plot shown in Fig. 7b that in either of the systems there is a definitive angular dependency exhibited by the PV current. For both systems studied, the normalized PV current fits the cosine function in (4) proving in this way that the origin of the PV current is the photogalvanic effect. However, we must take into consideration that equation (4) is calculated for rhombohedral symmetry. Therefore, in order to predict the exact response, which we obtain in lab coordinates, the BPV tensor must be transformed from rhombohedral to lab coordinates. We have performed this transformation for 71° domains. The details of this transformation are discussed in the Methods section. The net response obtained in the PLDW geometry can be expressed as flowing in the direction of both ferroelastic distortion and polarization, which is consistent with the theoretical results [16] . Similarly, the response in PPDW geometry can be expressed according to the equation From equation (5), we can observe that the current collected in PLDW geometry is composed of two components. The second term due to the BPV effect has a cosine dependency and will oscillate depending on angle θ . The first term is also due to the BPV effect but is independent of angle θ . This is also evident when we fit equation (5) to the data we measured in the PLDW geometry as shown in Fig. 7c . The θ -dependent behaviour of the BPV current is shifted by the non-oscillating first term of equation (5). The current in PPDW geometry has a sine dependency on angle θ . However, in order to compensate for the combined effects of factors such as misalignments between the electrodes and domains and a misalignment between the light beam direction and the normal to the sample surface, we have introduced a phase shift θ 0 and a constant current J 0 to equation (6), which now can be expressed as: From Fig. 7d , the agreement between the measured and predicted values from equation (7) is obvious. Based on equations (5, 6, 7) and the reported value of β 22 , we calculated the values of all the BPV coefficients, which are as follows β 15 =−7.1045 × 10 −5 V −1 , β 31 =−1.17 × 10 −4 V −1 and β 33 =9.74 × 10 −5 V −1 . Corresponding values of the glass coefficients are G 15 =−3.946 × 10 −10 cm V −1 , G 31 =−6.5 × 10 −10 cm V −1 and G 33 =5.41 × 10 −10 cm V −1 . We can now explain the scattered behaviour in the literature. The most important parameter seems to be the intrinsic conductivity. Samples in any form with high intrinsic conductivity should not show a large V oc . The high conductivity in BFO is a well-known problem, which might be the result of either unintentional doping of the raw material, or high oxygen vacancy density or any other fabrication parameter. Therefore, only the simple PV measurement at RT is not sufficient to conclude if a certain material exhibits the anomalous PV effect or not. A detailed complementary analysis of both dark conductivity and photoconductivity, including the temperature analysis and the spectral distribution of the latter (see Supplementary Figs S6 and S7 ), should be performed. In a thin film capacitor (plane-parallel) geometry, the film thickness is the most important parameter, as the open circuit voltage scales, according to equation (1), linearly with it. We would expect to obtain an open circuit voltage of about 0.6 Vμm −1 for the very favourable case shown in Fig 2a . Thus, to obtain a V oc larger than 3 V, the film thickness should be in the range of 5 μm. A large V oc in this geometry is not to be expected for usual sub-micron thicknesses. For a ceramic system, as the conductivity is extrinsic and usually through a grain boundary conduction mechanism, the value of V oc might depend tremendously on the effective fabrication process. Coming back to the role of the DW in the PV in BFO, we can state that the DW, due to their intrinsically higher conductivity, are rather detrimental for the abnormal PV effect. In normal cases and at room temperature, the only geometry, which allows high V oc values is that with the DW running parallel to the collecting electrodes. If the DW are contacting the two collecting electrodes, as in the perpendicular geometry, the expected V oc values are low, as the DW are acting rather as shunts. Nevertheless, the DW proved to show a markedly higher photoconductivity than the domain bulk. This means that the density of the non-equilibrium carriers generated at the DW is much higher than in the bulk, and this might be more significant for photoelectric devices based on BFO than the value of the open circuit voltage. In summary, by investigating the PV properties of BFO thin films in the low temperature range, it was observed that above-band-gap V oc (as large as 50 V) can be obtained irrespective of the domain wall geometry and the type of the domain wall. The V oc in all the samples and measurement geometries scaled up roughly exponentially with a decrease of temperature. The photogalvanic effect or the shift currents are at the origin of the abnormal PV effect in BFO. The high dark and photoconductivities of the DW are preventing a large open circuit voltage when these are connecting the collecting electrodes. Film growth Epitaxial BFO films of ~100 nm thickness were fabricated by pulsed laser deposition (PLD) technique. The films were deposited on orthorhombic TbScO 3 (110) oriented substrates at 650 °C with oxygen pressure of 0.145 mbar. The laser energy was 0.35 J cm −2 and the laser repetition rate was kept at 5 Hz. To fabricate films with 109° domains, the deposition was performed on bare TbScO 3 substrates. For obtaining 71° domains, the substrates were annealed in a tube furnace at 950 °C for 2 h along with an oxygen flow of ~200 sccm [1] , [25] . Piezoforce microscopy PFM was performed using a.c. excitation signal of 4 V amplitude and 33 kHz frequency applied on the AFM tip. AFM tips with Pt/Ti conductive coating and elastic constants of about 2 Nm −1 (NSC14, μMasch) were used. Photoelectric measurements The photoelectric effect was measured by illuminating the gap between the electrodes with a 405 nm ( hυ =3.06 eV) laser (Newport LQA405-85E) with a maximum power of 80 mW and simultaneously measuring the photocurrent using a high-input impedance electrometer (Keithley 6517). Variable temperature measurements were performed using an optical cryostat (Janis VPF-700). Open circuit voltage was extracted from the current voltage characteristics. BPV effect in ferroelectric materials BFO belongs to the space group R3c and many of the 27 elements of the third rank tensor will be reduced to zero owing to symmetry operations [26] , [27] , [28] , [29] . The tensor thereafter can be contracted into a 3 × 6 matrix of the form The incident light propagating along the Z -axis can be expressed as [28] , [29] The electric field vector E of the light can be resolved into two components along X and Y axes having cos θ and sin θ dependencies, respectively. Hence, where θ is the angle, which the polarization axis makes with the direction of current flow. As E is a second rank tensor, it can be expressed in the form of a 6 × 1 matrix and equation (3) takes the form [26] , [28] : From (11) we can approximate and Calculation of PV response The BPV tensor β ijk is a tensor of third rank. This means it has 3 3 elements. These elements can be expressed as: As the projections of the electric field vector of the light ( e j e k ) are symmetric with respect to each other, it means that the BPV tensor can be assumed to be symmetrical in j and k [27] , [29] . Due to this symmetry aspect, there remain only 18 independent coefficients, which can be conveniently represented in a matrix notation of the form: The coefficients in equation (12) are related to the coefficients in equation (13) in such an arrangement that the first suffix remains the same in both the notations, whereas the last two notations are related according to the relations presented in Table 1 (ref. 27 ): Table 1 Relation between matrix and tensor notation. Full size table However, there is a further reduction in the number of independent tensor coefficients due to the R3c symmetry of BFO. Henceforth, the matrix in equation (7) is reduced to [27] , [28] : It can be observed by comparing equation (13) and (14) that, β 22 = −β 21 = −β 16 , β 15 = β 24 and β 31 = β 32 (ref. 27 ). Therefore, the BPV effect in BFO can be completely described by the help of four independent coefficients, which are β 15 , β 22 , β 31 and β 33 . By using equation (14) and the matrix notations, we know that Based on the relations given in (15), we can rewrite equation (12) to obtain a third rank tensor, which would be valid for BFO: In order to predict the PV current, which we measure in lab coordinates, we must convert the BPV tensor from rhombohedral to lab coordinates. In addition, a film comprising of 71° domains, as shown in Supplementary Fig. S5 , consists of two kinds of rhombohedral unit cells, which results in two different domains. These have been shown as R-type and L-type in Supplementary Fig. S5 . Therefore, such a conversion must be performed for both the cells and domains. The matrices, which are required to transform the rhombohedral coordinate system of the R-and L-type domains to lab coordinates are given by [16] : The BPV tensor in the lab coordinates can then be expressed as a resultant of both the conversions: Based on the non-zero terms in equation (16), we can elaborate equation (19) as: From the relations given in (15) we can rearrange equation (20) to Having calculated the BPV tensor in lab coordinates, we can now predict the PV current in lab coordinates by The projections of the electric field of a linearly polarized light can be resolved into a second rank tensor via Jones matrix notation. This matrix can then be written in a (6 × 1) form of the type . Also, as explained previously, we can reduce the lab BPV tensor ( B qrs ) to a matrix notation of (3 × 6) type. Therefore, we can solve equation (22) by simple matrix multiplication with the result being of the type: As can be observed from equation (23), the main coefficients required to predict the PV current in PPDW and PLDW geometries are B 12 , B 16 , B 11 , B 22 , B 26 , B 21 . By substituting the values from equation (17) and (18) (using relation given in 15) into equation (21) we can calculate these terms to be: By substituting the values of the coefficients from equation (24)–(29), in equation (23), the calculated PV current in the parallel measurement geometry is Equation (30) can be further simplified by applying trigonometric operations resulting in The calculated PV current in the perpendicular measurement geometry is How to cite this article: Bhatnagar, A. et al. Role of domain walls in the abnormal photovoltaic effect in BiFeO 3 . Nat. Commun. 4:2835 doi: 10.1038/ncomms3835 (2013).